The dynamic relationships between the three events that release individual Na+ions from the Na+/K+-ATPase Na + /K + pumps move net charge through the cell membrane by mediating unequal exchange of intracellular Na + and extracellular K + . Most charge moves during transitions that release Na + to the cell exterior. When pumps are constrained to bind and release only Na + , a membrane voltage-step redistributes pumps among conformations with zero, one, two or three bound Na + , thereby transiently generating current. By applying rapid voltage steps to squid giant axons, we previously identified three components in such transient currents, with distinct relaxation speeds: fast (which nearly parallels the voltage-jump time course), medium speed ( τ m =0.2–0.5 ms) and slow ( τ s =1–10 ms). Here we show that these three components are tightly correlated, both in their magnitudes and in the time courses of their changes. The correlations reveal the dynamics of the conformational rearrangements that release three Na + to the exterior (or sequester them into their binding sites) one at a time, in an obligatorily sequential manner. The Na + /K + -ATPase ion pump, a member of the P-type family (named for their phosphorylated intermediates), harnesses the energy from hydrolysis of one ATP to alternately export three Na + and import two K + against their electrochemical gradients. By performing this active transport, the Na + /K + pump has an essential role in the homeostasis of intracellular Na + and K + , crucial to sustaining cell excitability, volume and Na + -dependent secondary transport. On the basis of biochemical data accumulated during the decade following its discovery [1] , the Na + /K + -ATPase was proposed to transport Na + and K + ions according to a model known as the Post-Albers scheme [2] , [3] ( Fig. 1 ). As ions are transported through the Na + /K + pump, they become temporarily occluded within the protein, inaccessible (symbolized by parentheses) from either cytoplasmic or extracellular side of the membrane, before being released [4] , [5] , [6] , [7] . By working in the absence of intracellular and extracellular K + , but presence of intracellular ATP, thereby effectively restricting Na + /K + pumps to the reversible transitions associated with deocclusion/occlusion and extracellular release/binding of Na + (conformations encompassed by the dotted box in Fig. 1 ), Nakao and Gadsby [8] were able to detect presteady-state electrical signals accompanying those transitions in response to steps of membrane potential. The signals arise because Na + ions traverse a fraction of the transmembrane electric field as they enter or leave their binding sites deep within the pump [9] , [10] , [11] , [12] , [13] . At a given membrane potential and external sodium concentration ([Na + ] o ), the populations of pumps with empty binding sites, and those with bound or occluded Na + (that is, dotted box conformations, Fig. 1 ), reach a steady-state distribution. A sudden change of membrane voltage then shifts the Na + -binding equilibrium, and initiates a redistribution of the pump populations towards a new steady-state arrangement. The consequent change in Na + -binding-site occupancy causes Na + ions to travel between the extracellular environment and the pump interior, through the electric field, so generating current. As the new steady distribution is approached, fewer Na + ions move, and the current declines. The electrical signals therefore appear as transient currents. 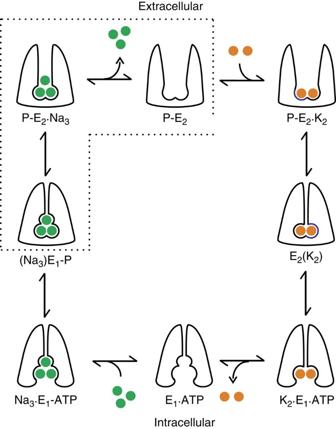Figure 1: Post-Albers diagram of the Na+/K+transport cycle. In this simplified scheme, E1conformations represent those in which binding sites may be accessed from the intracellular side. In these states, two K+(orange balls) are released, three Na+(green balls) are bound and occluded, and the protein is phosphorylated. In P-E2conformations, the binding sites become accessible from the external environment, and the three Na+are released, two K+are bound and occluded, and the protein autodephosphorylates. The states enclosed by the dotted box were isolated by removal of K+from all solutions and by the presence of 5 mM MgATP (and of ADP scavengers)8,14in the internal solution. Figure 1: Post-Albers diagram of the Na + /K + transport cycle. In this simplified scheme, E 1 conformations represent those in which binding sites may be accessed from the intracellular side. In these states, two K + (orange balls) are released, three Na + (green balls) are bound and occluded, and the protein is phosphorylated. In P-E 2 conformations, the binding sites become accessible from the external environment, and the three Na + are released, two K + are bound and occluded, and the protein autodephosphorylates. The states enclosed by the dotted box were isolated by removal of K + from all solutions and by the presence of 5 mM MgATP (and of ADP scavengers) [8] , [14] in the internal solution. Full size image By exploiting the ability of axial current delivery in the squid giant axon to very rapidly step membrane voltage, we previously identified three phases of relaxation of transient pump currents [11] : fast (comparable to the voltage-jump time course), medium speed ( τ m =0.2–0.5 ms) and slow ( τ s =1–10 ms). We suggested that each phase reflects a distinct Na + -binding (or release—depending on voltage change direction) event with its associated conformational transition (occlusion or deocclusion). Now, marked technical advances have allowed us to follow the amounts of charge moved in all three phases, simultaneously, with unprecedented temporal resolution. We show that, over a broad range of [Na + ] o and membrane potential, regardless of when the voltage-step assay is initiated, the amount of charge moved by the fast component is dictated by the status of the medium-speed component at that time, which is itself determined by the extant status of the slow component. Thus, under all conditions examined, as Na + -bound and unbound pump populations redistribute, the amounts and time courses of the three charge movements are closely correlated. These strict correlations elucidate the dynamic relationships between the successive steps that bind or release the three Na + ions at the Na + /K + pump's extracellular surface. Pump-mediated charge movement We obtained Na + /K + pump current as the component of membrane current inhibited by 50–100 μM dihydrodigitoxigenin (H 2 DTG), a specific and reversible squid Na + /K + pump inhibitor [14] that, similar to other cardiotonic steroids, immobilizes Na + /K + pumps in a P-E 2 (Na 2 ) state [15] . 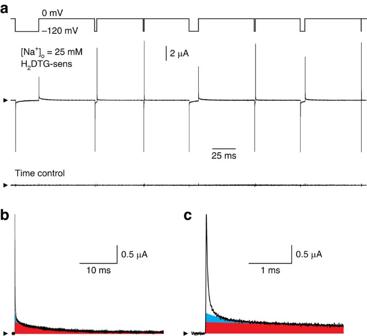Figure 2: Pump-mediated transient currents at 25 mM [Na+]o. (a) Voltage protocol, H2DTG-sensitive current and time control. The voltage protocol (upper trace) comprised seven voltage steps from 0 to −120 mV, with durations of 25, 2, 0.5, 10, 1, 5 and 0.1 ms. Pump-mediated current (middle trace) was determined by subtracting membrane current obtained in the presence of H2DTG from the current record acquired 40 s earlier, before the inhibitor was added. The time control record (lower trace) reflects any changes in membrane current during the 40-s period immediately preceding H2DTG application. Arrowheads (also inb,c) indicate zero current. (b) Pump-mediated transient current on return to 0 mV at the end of the first (25-ms) voltage step. The red area denotesQscharge. (c) Time axis expansion ofb. The cyan area representsQmcharge. These two components were quantified from the time constants and amplitudes of extrapolated zero-time intercepts of a two-exponential fit begun 500 μs after the voltage step back to 0 mV. Subtracting this fit from the entire transient current yieldedQfcharge (white area). Figure 2a (middle trace) shows H 2 DTG-sensitive (that is, pump-mediated) current, determined in an axon exposed to 25 mM [Na + ] o and 0 [K + ] o , in response to a voltage protocol (top trace) that comprised a sequence of seven voltage jumps, from 0 to −120 mV for varying durations. Each step to −120 mV elicited a large fast component of pump-mediated charge movement ( Q f ) of the same magnitude, verifying that all seven voltage steps began from the same initial conditions, that is, steady state at 0 mV. Q f relaxation at −120 mV was only slightly slower than the membrane voltage change, consistent with Q f reflecting Na + ions moving from the bulk solution though part of the membrane's electric field to their binding sites deep in the protein ( Fig. 1 ; top left). Almost immediate return of the membrane potential to 0 mV (for example, after the seventh, briefest, step to −120 mV) caused a fast pump-mediated charge movement of similar size and speed, but opposite sign, consistent with discharge back to the bulk solution of all Na + that had just entered pump binding sites at −120 mV. Figure 2: Pump-mediated transient currents at 25 mM [Na + ] o . ( a ) Voltage protocol, H 2 DTG-sensitive current and time control. The voltage protocol (upper trace) comprised seven voltage steps from 0 to −120 mV, with durations of 25, 2, 0.5, 10, 1, 5 and 0.1 ms. Pump-mediated current (middle trace) was determined by subtracting membrane current obtained in the presence of H 2 DTG from the current record acquired 40 s earlier, before the inhibitor was added. The time control record (lower trace) reflects any changes in membrane current during the 40-s period immediately preceding H 2 DTG application. Arrowheads (also in b , c ) indicate zero current. ( b ) Pump-mediated transient current on return to 0 mV at the end of the first (25-ms) voltage step. The red area denotes Q s charge. ( c ) Time axis expansion of b . The cyan area represents Q m charge. These two components were quantified from the time constants and amplitudes of extrapolated zero-time intercepts of a two-exponential fit begun 500 μs after the voltage step back to 0 mV. Subtracting this fit from the entire transient current yielded Q f charge (white area). Full size image But, during the longer voltage steps (for example, the first in the sequence), the rapid initial charge movement at −120 mV was eventually followed by a much slower, and lower-amplitude, current decay representing the slow charge component ( Q s ) linked to the major occlusion transition P-E 2 .Na 3 ↔(Na 3 )E 1 -P ( Fig. 1a ). The longest steps to −120 mV allow the distribution of pumps to attain a new steady state, poised towards the occluded conformation (Na 3 )E 1 -P. In those cases, return of the membrane potential to 0 mV elicited not only a rapidly decaying, though relatively low amplitude, outward Q f , reflecting release of bound Na + from P-E 2 .Na 3 , but also a subsequent slowly decaying Q s , reflecting deocclusion and release through the electric field of Na + that had become occluded in (Na 3 )E 1 -P at −120 mV. Because, on return to 0 mV, Na + ions occluded at −120 mV must await deocclusion before they can be released to the bulk solution, the quantity of Na + released immediately ( Q f ) showed a strong inverse correlation with step duration; the longer the stay at −120 mV, the smaller the amplitude of the rapidly decaying current on return to 0 mV ( Fig. 2a ). We showed previously that such pump-mediated presteady-state currents comprise at least three components [11] , readily distinguished and separated when the voltage is stepped back to 0 mV ( Fig. 2b,c ). After the long sojourn at −120 mV, by far, the largest proportion of the charge (area underneath the transient current trace) was carried by the slow component ( Fig. 2b , red area; fitted time constant at 0 mV, τ s =8.40±0.01 ms), which was preceded by at least two faster-decaying components ( Fig. 2c , cyan and white areas; see also Fig. 3a ). The slower of these, the medium-speed component ( Q m , cyan; fitted time constant at 0 mV, τ m =0.55±0.03 ms), was considerably (>10-fold) slower than the change in axon membrane potential, whereas the decay of the fast component of pump charge ( Q f , white) was comparable with the speed of the voltage jump (given by the slowest part of the membrane capacitance current decay; τ =28.0±0.3 μs; Supplementary Fig. S1 ). 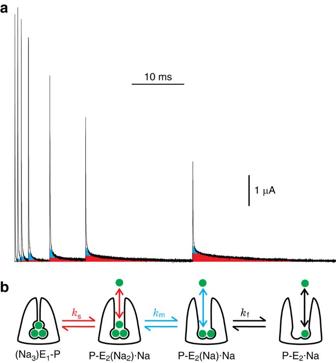Figure 3: Distinct changes of the three charge components and scheme symbolizing binding/release and occlusion/deocclusion of three external Na+by the Na+/K+pump. (a) Superposition of the current decays at 0 mV following each of the seven voltage steps inFigure 2a, after aligning the traces to the initial jump to −120 mV; for clarity, the first 0.1 ms of all records, and all currents <0, have been omitted from the figure. With longer stays at −120 mV,Qs(red) increased monotonically, whereasQm(cyan) andQf(white) initially increased but then declined. (b) External Na+ions (green) are modelled as interacting with the pump in three distinct, sequential, binding/release events each associated with a conformational transition that rate limits the corresponding charge component, slow (red), medium speed (cyan) or fast (black). Figure 3: Distinct changes of the three charge components and scheme symbolizing binding/release and occlusion/deocclusion of three external Na + by the Na + /K + pump. ( a ) Superposition of the current decays at 0 mV following each of the seven voltage steps in Figure 2a , after aligning the traces to the initial jump to −120 mV; for clarity, the first 0.1 ms of all records, and all currents <0, have been omitted from the figure. With longer stays at −120 mV, Q s (red) increased monotonically, whereas Q m (cyan) and Q f (white) initially increased but then declined. ( b ) External Na + ions (green) are modelled as interacting with the pump in three distinct, sequential, binding/release events each associated with a conformational transition that rate limits the corresponding charge component, slow (red), medium speed (cyan) or fast (black). Full size image Temporal correlations between the three charge components We interpreted [11] the three components of transient pump current as representing movements of the three Na + in and out of the Na + /K + -ATPase ( Fig. 3b ), each rate-limited by a linked occlusion/deocclusion transition. Such a model predicts that changes in the three components on shifting from one steady-state distribution to another must be correlated. To test that prediction, we have now tracked the quantity of charge carried by each individual component as the duration of the −120 mV step was prolonged ( Figs 2a and 3a ). The progression from the initial steady state at 0 mV towards the final steady state at −120 mV was followed by assaying, after various times spent at −120 mV (100 μs–25 ms in the experiment of Figs 2a and 3a ), the quantity of each charge component that moved back during reestablishment of the original steady state at 0 mV. The amounts of slow- and medium-speed charge, Q s and Q m , were determined as products of the time constants and amplitudes (the time zero intercepts) derived from two-exponential fits to the current decaying at 0 mV, the fits beginning 400–600 μs after the step back to 0 mV. To determine the amount of Q f charge, each two-exponential fit was subtracted from its corresponding complete transient pump current record, and the remainder (white areas enclosed by current traces in Figs. 2c and 3a ) was numerically integrated, and then corrected for any time-control error; examples of these small errors are seen in the time-control traces of Figure 2a and Supplementary Figure S2 . The sizes of the three components of charge assayed at 0 mV after each visit to −120 mV were all normalized to the Q s -value obtained following the longest stay there, and the results were plotted against the time spent at −120 mV ( Fig. 4a–c ). 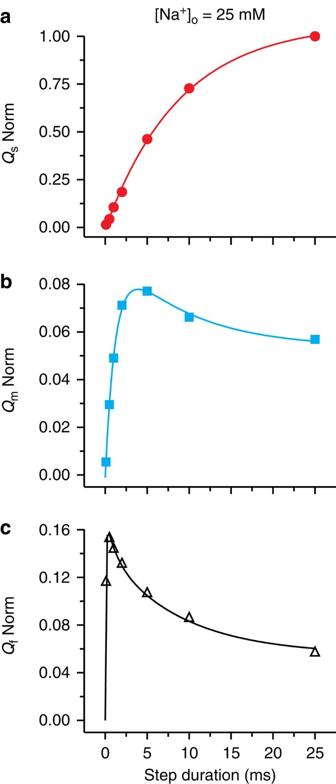Figure 4: Charge movements measured in a single axon at 0 mV and 25 mM [Na+]oreport on time courses and sequences of events at −120 mV. (a)Qsincreased monotonically towards a maximum value with the duration of the preceding stay at −120 mV; the magnitude ofQsafter the 25-ms stay at −120 mV was used to normalize other charge components. The solid red line shows an exponential fit toQswithτs=8.9±0.4 ms. (b)Qmincreased quickly with a fittedτm=1.2±0.1 ms (cyan curve) before decaying with a time course that was well described byτs(here fixed at 8.9 ms). (c)Qfdeveloped very rapidly (<0.5 ms) and then decayed (black curve) with a biexponential time course well described by time constantsτmandτs(here fixed at 1.2 and 8.9 ms, respectively). Figure 4: Charge movements measured in a single axon at 0 mV and 25 mM [Na + ] o report on time courses and sequences of events at −120 mV. ( a ) Q s increased monotonically towards a maximum value with the duration of the preceding stay at −120 mV; the magnitude of Q s after the 25-ms stay at −120 mV was used to normalize other charge components. The solid red line shows an exponential fit to Q s with τ s =8.9±0.4 ms. ( b ) Q m increased quickly with a fitted τ m =1.2±0.1 ms (cyan curve) before decaying with a time course that was well described by τ s (here fixed at 8.9 ms). ( c ) Q f developed very rapidly (<0.5 ms) and then decayed (black curve) with a biexponential time course well described by time constants τ m and τ s (here fixed at 1.2 and 8.9 ms, respectively). Full size image As evident in the current traces of Figure 3a and in the graph of Figure 4a (which summarize data from a single axon), the magnitude of Q s (red) observed at 0 mV rose mono-exponentially with time spent at −120 mV, yielding a τ s of 8.9±0.4 ms ( Fig. 4a ), characteristic of the occlusion transition, P-E 2 (Na 2 )·Na↔(Na 3 )E 1 -P ( Fig. 3b , left), at −120 mV after the third Na + has bound [11] . Q m (cyan) from the same axon exhibited a biphasic time course ( Figs 3a and 4b ), initially increasing with time spent at −120 mV with τ m =1.2±0.1 ms, but then decaying along a time course that was well fit by τ s (8.9 ms). Q f (white area, black fit curve) from the same experiment also displayed a biphasic time course ( Figs 3a and 4c ), but with a rapid increase followed by a biexponential decay whose time constants corresponded to τ m (1.2 ms) and τ s (8.9 ms). Interestingly, the amounts of Q m and Q f never exceeded a small fraction of Q s (at 25 mM [Na + ] o , peak Q m and Q f averaged 7±1 and 14±1% ( n =8), respectively, of the largest Q s ), and were even smaller after a near steady state was reached at −120 mV (steady Q m amounted to only 4±1%, and Q f to 3±1% ( n =8) of Q s after the longest step). Dependence of the three charge components on extracellular Na + Increasing [Na + ] o accelerated the ascending phase of all three components ( Fig. 5a,b ), providing support for the interpretation that each component reflects a distinct Na + binding/release event. As shown for 25 mM [Na + ] o above ( Fig. 4 ), in both 50 mM ( Fig. 5a ) and 400 mM [Na + ] o ( Fig. 5b ), the time course of the decay of Q m was well described by τ s . Similarly, at each [Na + ] o , the decay of Q f was biexponential with time constants corresponding to the respective τ m and τ s . In addition, the relative amplitudes of Q m and Q f charge movements on jumping back to 0 mV after attaining a near steady state at −120 mV, as a proportion of their peak magnitudes after shorter stays there, were smaller at higher [Na + ] o ( Fig. 5 ; Supplementary Fig. S2 ). 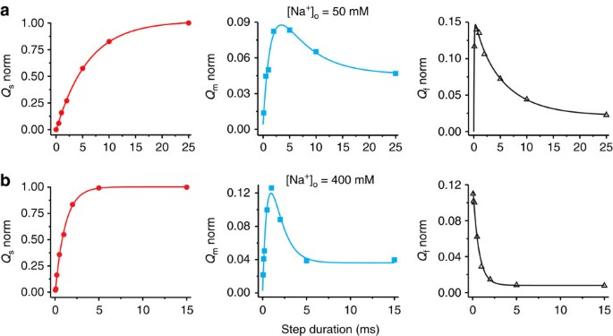Figure 5: [Na+]odependence of the time courses and amplitudes of the three charge components. Colour and symbol coding, as well as bases for solid line fits, are as inFigure 4. (a) Data from a single axon at 50 mM [Na+]o: fittedτs=6.0±0.2 ms,τm=1.5±0.3 ms. (b) A different axon at 400 mM [Na+]o: fittedτs=1.1±0.1 ms,τm=0.65±0.10 ms. Figure 5: [Na + ] o dependence of the time courses and amplitudes of the three charge components. Colour and symbol coding, as well as bases for solid line fits, are as in Figure 4 . ( a ) Data from a single axon at 50 mM [Na + ] o : fitted τ s =6.0±0.2 ms, τ m =1.5±0.3 ms. ( b ) A different axon at 400 mM [Na + ] o : fitted τ s =1.1±0.1 ms, τ m =0.65±0.10 ms. Full size image Full mechanistic understanding of the series of conformational transitions that underlie alternate binding and transport of Na + and K + ions by the Na + /K + pump ( Fig. 1 ) requires a combination of structural information at high spatial resolution and dynamic information at high temporal resolution. To obtain precise kinetic information, the transport cycle must be restricted to a tractable subset of transitions. In this work, we limited pumps to the extracellular Na + release/binding transitions (dotted box in Fig. 1 ) by working in the absence of internal and external K + , but presence of intracellular ATP. Previous results established that most of the charge movement, and hence voltage dependence, of the transport cycle arises within these transitions [8] , [16] , [17] as Na + ions travel to and from their binding sites along narrow access channels through part of the electric field [9] , [10] , [11] , [18] . Here we studied the relationships between the individual release/binding transitions of extracellular Na + in native Na + /K + pumps of internally dialysed squid giant axons, which allow both intra- and extracellular environments to be controlled reliably, and membrane voltage to be changed rapidly. We previously identified three phases of charge movements during interactions of extracellular Na + with squid axon Na + /K + pumps [11] , fast, medium speed and slow, each of which we suggested reflected binding or release of one of the three Na + . We found a reciprocal relationship between the sizes of the medium speed and slow components that suggested that those events occurred in sequence. But our measurements lacked the precision to discern whether the fast component also occurred in sequence with the medium-speed component. It remained possible, therefore, that two Na + are released/bound sequentially, but that movement of the third Na + represents a kinetically distinct, parallel process. By improving our axon superfusion and data acquisition systems, we have now been able to establish the temporal relationships and absolute magnitudes of changes in all three components (for example, Fig. 3a ), at the same time, with previously unattainable precision. We found that the amount of Q s measured at 0 mV developed monotonically towards a maximum as the preceding step to negative potentials was prolonged ( Figs 3a , 4a and 5 ). At all [Na + ] o , the time constant of that rise, τ s (averaging 7.9±0.3 ( n =7), 5.6±0.2 ( n =7) and 1.5±0.1 ( n =12) ms, respectively, at 25, 50 and 400 mM [Na + ] o ) mirrored the slow relaxation of the transient current (average τ of 7.9±0.5 ( n =13), 5.5±0.2 ( n =6) and 1.3±0.1 ( n =10) ms, respectively) at the negative conditioning potential (−120 or −140 mV; −120 mV illustrated here), rather than the slow current relaxation at 0 mV (average τ of 9.7±0.3 ( n =14), 9.4±0.3 ( n =7) and 5.8±0.2 ( n =13) ms, respectively). As the slowly decaying current at negative voltages reports accumulation of the occluded conformation, (Na 3 )E 1 -P, following binding of the third Na + (refs 8 , 9 , 10 , 11 , 12 , 13 and 16 ), we can conclude that (Na 3 )E 1 -P occupancy determines the quantity of Q s observed at 0 mV, which thus reflects release of the first Na + from P-E 2 (Na 2 )·Na, rate-limited by the deocclusion transition, (Na 3 )E 1 -P↔P-E 2 (Na 2 )·Na ( Fig. 3b , left). In contrast to this monotonic trajectory for Q s , the development of both Q m and Q f (assayed, similar to Q s , at 0 mV) as a function of time spent at the negative conditioning voltage was biphasic. In both cases, after initially increasing, the charge eventually diminished with a time course that matched τ s , indicating that sequestration of pumps in the occluded (Na 3 )E 1 -P state precluded their contributing to Q m or Q f charge on return to 0 mV. The events generating Q m and Q f are therefore each in series with the occlusion/deocclusion step that gives rise to Q s . The mono-exponential relaxation of Q m with time constant equivalent to τ s argues that the Q m -generating transition lies, kinetically, adjacent to the (Na 3 )E 1 -P↔P-E 2 (Na 2 )·Na step. The additional fact that Q f relaxed biexponentially with time constants that reflect τ m and τ s argues that the transition associated with Q f is adjacent to that generating Q m . We can conclude, then, that the transition that generates Q m is sandwiched between the transition associated with Q s and that associated with Q f . Given the three separable charge components, the three distinct time constants, and the expectation that three Na + become occluded at negative potentials, the most parsimonious scheme to account for these results is that shown in Figure 3b . This model depicts strictly sequential binding or release of one Na + at a time (coloured vertical arrows) through a fraction of the membrane's electric field, each Na + ion giving rise to a transient current component with a time course governed (coloured horizontal arrows) by the subsequent occlusion step in the case of negative voltage jumps, or by the preceding deocclusion in the case of positive voltage jumps. According to this scheme, a step from a negative potential to 0 mV will elicit fast, medium speed and slow outward transient charge components with magnitudes dictated, respectively, by the occupancies of states P-E 2 (Na), P-E 2 (Na 2 ) and (Na 3 )E 1 -P at the instant the step is initiated. It is the changes in occupancies of those states during the time spent at −120 mV that are mirrored in the curves in Figures 4 and 5 . The sensitivity to [Na + ] o of the time courses of all three charge components ( Figs 4 and 5 ), and hence of the occupancies of all three states, further supports the existence of three separate external Na + -binding steps. If each component indeed reflects motion of a single Na + ion through part of the electric field on entering or leaving its binding site, the relatively small [9] peak magnitudes of Q m and Q f —only 7–14% of the largest Q s , over the full 25–400 mM range of [Na + ] o examined—can now be confidently attributed to weaker electrogenicity of the last two Na + -ion release steps; this likely reflects the relatively wide extracellular access pathway, and hence weakened electric field, expected at least for the P-E 2 state, from which the final Na + ion is released, based on the E 2 ·BeF 3 − Ca 2+ -ATPase crystal structure [19] , [20] . These findings shed new light on the stepwise structural changes that progressively open the extracellular access pathway in the Na + /K + pump, a model P-type ATPase. Solutions Giant axons from the squid Loligo pealei were internally dialysed and externally superfused at 21–23°C with solutions devised to distribute Na + /K + pumps among Na + deocclusion/release transitions ( Fig. 1 , enclosed by dotted box). The intracellular solution contained (in mM): 80 Na-HEPES, 57 N -methyl- D -glucamine-HEPES, 50 glycine, 50 phenylpropyltriethyl-ammonium sulphate (to block potassium channels), 5 dithiothreitol, 2.5 BAPTA, 15 Mg-HEPES, 5 Tris-ATP, 5 phospho(enol) pyruvate tri-Na + salt and 5 phospho- L -arginine mono-Na + salt (pH 7.6, adjusted with HEPES). The composition of the extracellular solution was (in mM): 400 Na-sulphamate, 75 Ca 2+ -sulphamate, 1 3,4-diaminopyridine, 2×10 −4 tetrodotoxin, 5 Tris-HEPES and 0.05 EDTA (pH 7.7, adjusted with N -methyl- D -glucamine or sulphamic acid). Na-sulphamate was replaced by tetramethylammonium-sulphamate in solutions containing lower external Na + concentrations. Osmolality of all solutions was ∼ 930 mOsmol kg −1 . In principle, these experimental solutions could support uncoupled Na + efflux [21] , a non-canonical mode of Na + /K + pump operation that occurs several orders of magnitude more slowly than the slowest Na + occlusion/deocclusion step, and so could not affect our measurements. Electrophysiology Voltage steps were generated and currents recorded using a 14-bit high-speed AD/DA conversion board (A4D1, Innovative Integration) with software developed in-house. Currents were filtered at 100–150 kHz with an 8-pole Bessel filter (Frequency Devices 90IP), then sampled at 1 MHz. Na + /K + pump current was resolved as current sensitive to H 2 DTG, a specific and reversible inhibitor of the squid pump [14] . Pump currents were analysed with in-house software and OriginLab v8. To study the temporal correlations between the individual components of pump-mediated current, the experimental system must remain nearly perfectly stable. Because pump currents are obtained by subtracting membrane current traces acquired before and after H 2 DTG addition, any alteration of other electrical properties of the system during that time interval would preclude meaningful interpretation of the subtracted current. For example, changes in series resistance, presumably due to changes in the Frankenhäuser-Hodgkin space surrounding the axon, are known to occur over time [22] . So we redesigned our superfusion system to speed the action of H 2 DTG ( τ now ∼ 7 s; Supplementary Fig. S3 ) and time-control errors are now diminished, as evident from the time control-traces similar to those in Figure 2a and Supplementary Figure S2 . An additional technical improvement is a more powerful acquisition system that allows an entire experiment to be captured in a single record while maintaining the high temporal resolution of ≥1 MHz sampling. How to cite this article: Gadsby, D.C. et al . The dynamic relationships between the three events that release individual Na + ions from the Na + /K + -ATPase. Nat. Commun. 3:669 doi: 10.1038/ncomms1673 (2012).